Local membrane charge regulates β2adrenergic receptor coupling to Gi3 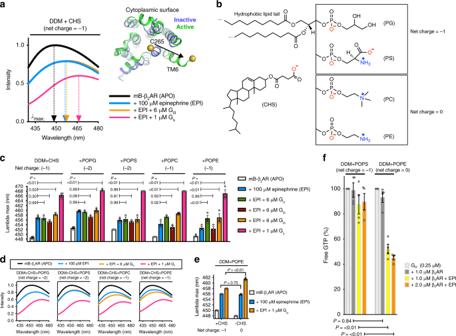Fig. 1 Negatively charged lipids inhibit β2AR−Gicoupling in detergent.amB−β2AR emission spectra in DDM + CHS micelles (5:1 DDM:CHS mole ratio) in the absence of epinephrine (APO) and in the presence of epinephrine, ± G protein (Gsor Gi3). Arrows point to the lambda max value, i.e. the wavelength where mB emission intensity is greatest. Inset shows how Gscoupling alters the structure of mB−β2AR, highlighting the change in position of monobromobimane (mB) at C265 of transmembrane 6 (TM6) (Inactive: PDB 5JQH74; Active: PDB 3SN669).bStructures of CHS and phospholipids, with net charge indicated.cEffect of phospholipid on mB−β2AR interaction with G protein (Gi1, Gi2, Gi3, and Gs), read out as an increase in lambda max. Interaction was assessed in the absence of lipid (5:1 DDM:CHS mole ratio) and in the presence of POPG, POPS, POPC, or POPE (5:1:1 DDM:CHS:Lipid mole ratio). Multiplicity adjustedPvalues were computed by two-way ANOVA followed by Dunnett’s post hoc test between indicated groups.dSelected mB−β2AR emission spectra from panel (c).eEffect of CHS on mB−β2AR interaction with 1 μM Gi3. Interaction was assessed in the presence of CHS (5:1:1 DDM:POPE:CHS mole ratio) or in the absence of CHS (5:1 DDM:POPE mole ratio). Multiplicity adjustedPvalues were computed by two-way ANOVA followed by Sidak’s post hoc test between indicated groups.a–emB−β2AR concentration is 300 nM. Data are mean of three independent experiments.fβ2AR-induced GTP turnover for Gi3(± 200 μM epinephrine, EPI) in DDM + POPS (5:1 DDM:POPS mole ratio) and in DDM + POPE (5:1 DDM:POPE mole ratio). Free GTP was assayed after 12 min. Luminescence signals were normalized relative to the condition with Gi3alone (see Supplementary Fig.4). Data are mean ± s.e.m. of four independent experiments. Multiplicity adjustedPvalues were computed by two-way ANOVA followed by Sidak’s post hoc test between indicated groups. Source data are provided in the Source Data File The β 2 adrenergic receptor (β 2 AR) signals through both G s and G i in cardiac myocytes, and the G i pathway counteracts the G s pathway. However, G i coupling is much less efficient than G s coupling in most cell-based and biochemical assays, making it difficult to study β 2 AR−G i interactions. Here we investigate the role of phospholipid composition on G s and G i coupling. While negatively charged phospholipids are known to enhance agonist affinity and stabilize an active state of the β 2 AR, we find that they impair coupling to G i3 and facilitate coupling to G s . Positively charged Ca 2+ and Mg 2+ , known to interact with the negative charge on phospholipids, facilitates G i3 coupling. Mutational analysis suggests that Ca 2+ coordinates an interaction between phospholipid and the negatively charged EDGE motif on the amino terminal helix of G i3 . Taken together, our observations suggest that local membrane charge modulates the interaction between β 2 AR and competing G protein subtypes. A third of all FDA-approved pharmaceutical drugs function by modulating the activity of G-protein-coupled receptors (GPCRs) [1] , a large receptor superfamily. GPCRs catalyze the activation of heterotrimeric G proteins, which in turn initiate a multitude of signaling cascades that alter cellular function. The β 2 adrenergic receptor (β 2 AR) is a prototypical GPCR that mediates the fight-or-flight response. β 2 AR signals through both G s and G i , and the dual G protein selectivity of β 2 AR is best characterized in heart muscle (cardiac myocytes). In healthy neonatal cardiac myocytes, epinephrine-stimulated β 2 AR immediately activates G s , increasing contraction rate, but after 10−15 min β 2 AR signals predominantly through G i [2] , which decreases the contraction rate. In cardiac myocytes, β 2 AR couples to both G i2 and G i3 [3] . Of interest, G i activation is impaired if β 2 AR internalization is blocked [4] . Also, G i does not interact with a modified β 2 AR that internalizes but does not recycle to the plasma membrane [5] , or with WT β 2 AR that internalizes but is pharmacologically blocked from recycling [6] . Taken together, these observations demonstrate that β 2 AR−G i interaction is regulated temporally and perhaps spatially. During heart failure, a condition of chronic, progressive cardiac insufficiency, the G i pathway counteracts some negative consequences of chronic G s activation that exacerbate heart failure, namely apoptosis and structural and functional remodeling [7] , [8] , [9] . However, G i activation reduces contractility, which can be problematic in certain models of heart failure [10] . More precise regulation of G s and G i activation is a therapeutic aim [9] . While β 2 AR signals through both G s and G i , the mechanism that initiates the G s -to-G i switch in the healthy heart is not fully understood. Multiple biochemical mechanisms may play a role. PKA phosphorylation of β 2 AR has been reported to increase G i1 coupling in vitro [11] and G i coupling in HEK cells [12] ; however, the G i1 subtype is not expressed in cardiac myocytes, and β 2 AR−G i coupling is PKA independent in these cells [2] . In addition, GRK2 phosphorylation of β 2 AR has been suggested to increase G i coupling [13] , but other investigators have reported that dephosphorylation is critical for β 2 AR recycling to the plasma membrane, and β 2 AR−G i interactions [6] . Therefore, the mechanisms that modulate β 2 AR−G i coupling remain unclear. In vitro, negatively charged phospholipids stabilize an active conformation of the β 2 AR and enhance its affinity for the catecholamine isoproterenol [14] , but the effect of phospholipid charge on G protein coupling is unknown. Negatively charged lipids have previously been shown to facilitate β 1 AR−G s interaction [15] , NTS1−G q [16] interaction, CB 2 −G protein interaction [17] , and rhodopsin−G t [18] interaction. In cardiac myocytes, β 2 AR activates G s in T-tubules [19] , deep evaginations of the plasma membrane enriched in L-type calcium channels and negatively charged phospholipids [20] . β 2 AR activation of G i may also occur in T-tubules, after internalization and recycling. However, trafficking events may alter the composition of phospholipids surrounding the β 2 AR. In addition, the β 2 AR−G s signaling that occurs prior to β 2 AR−G i signaling greatly increases the Ca 2+ concentration near T-tubules [21] , which may alter the charge properties of the T-tubule lipids [22] . Here we examine the effect of phospholipid charge on β 2 AR interactions with G s and G i3 . We find that negatively charged lipids enhance β 2 AR interaction with G s and impair interaction with G i3 . Further, Ca 2+ and Mg 2+ facilitate β 2 AR−G i3 interaction in negatively charged lipids. Our observations suggest that local membrane charge, tuned by intracellular cations, modulates β 2 AR interaction with G i3 . Monitoring G protein coupling by fluorescence spectroscopy Epinephrine activates β 2 AR by partially stabilizing the conformation recognized by the G protein. This conformation is fully stabilized upon G protein coupling [23] , [24] , [25] . A feature of the G-protein-coupled conformation of β 2 AR is a 14 angstrom outward displacement of the cytoplasmic end of β 2 AR transmembrane segment 6 (TM6) (Fig. 1a ). This conformation can be detected by fluorescence spectroscopy, using a modified β 2 AR labeled at the cytoplasmic end of TM6 with an environmentally sensitive fluorophore, monobromobimane (mB−β 2 AR, see Methods and ref. [26] ). Outward movement of TM6 affects the environmental polarity of mB, going from the hydrophobic receptor core to the solvent, decreasing the intensity of mB and increasing the wavelength where emission intensity is greatest ( λ max ), from ~447 to ~468 nm (Fig. 1a ). We monitor λ max to detect G protein coupling, as λ max increases with coupling (Supplementary Fig. 1 ). Fig. 1 Negatively charged lipids inhibit β 2 AR−G i coupling in detergent. a mB−β 2 AR emission spectra in DDM + CHS micelles (5:1 DDM:CHS mole ratio) in the absence of epinephrine (APO) and in the presence of epinephrine, ± G protein (G s or G i3 ). Arrows point to the lambda max value, i.e. the wavelength where mB emission intensity is greatest. Inset shows how G s coupling alters the structure of mB−β 2 AR, highlighting the change in position of monobromobimane (mB) at C265 of transmembrane 6 (TM6) (Inactive: PDB 5JQH [74] ; Active: PDB 3SN6 [69] ). b Structures of CHS and phospholipids, with net charge indicated. c Effect of phospholipid on mB−β 2 AR interaction with G protein (G i1 , G i2 , G i3 , and G s ), read out as an increase in lambda max. Interaction was assessed in the absence of lipid (5:1 DDM:CHS mole ratio) and in the presence of POPG, POPS, POPC, or POPE (5:1:1 DDM:CHS:Lipid mole ratio). Multiplicity adjusted P values were computed by two-way ANOVA followed by Dunnett’s post hoc test between indicated groups. d Selected mB−β 2 AR emission spectra from panel ( c ). e Effect of CHS on mB−β 2 AR interaction with 1 μM G i3 . Interaction was assessed in the presence of CHS (5:1:1 DDM:POPE:CHS mole ratio) or in the absence of CHS (5:1 DDM:POPE mole ratio). Multiplicity adjusted P values were computed by two-way ANOVA followed by Sidak’s post hoc test between indicated groups. a – e mB−β 2 AR concentration is 300 nM. Data are mean of three independent experiments. f β 2 AR-induced GTP turnover for G i3 (± 200 μM epinephrine, EPI) in DDM + POPS (5:1 DDM:POPS mole ratio) and in DDM + POPE (5:1 DDM:POPE mole ratio). Free GTP was assayed after 12 min. Luminescence signals were normalized relative to the condition with G i3 alone (see Supplementary Fig. 4 ). Data are mean ± s.e.m. of four independent experiments. Multiplicity adjusted P values were computed by two-way ANOVA followed by Sidak’s post hoc test between indicated groups. Source data are provided in the Source Data File Full size image Negatively charged lipids inhibit β 2 AR-G i coupling In the presence of epinephrine, we observe a change in intensity and λ max of mB−β 2 AR following the addition of G s in a detergent mixture containing n -dodecyl-β- d -maltopyranoside (DDM) and cholesteryl hemisuccinate (CHS) that is commonly used for biochemical study of GPCR/G protein complexes (Fig. 1a ). In contrast, the coupling efficiency of mB−β 2 AR−G i3 was relatively weak (Fig. 1a ). Next, we compared the coupling efficiency of mB−β 2 AR−G i in DDM + CHS mixtures with different phospholipids incorporated (Fig. 1b–d ). While we were unable to detect interactions of mB−β 2 AR with G i1 , G i2 or G i3 in the presence of negatively charged lipids phosphatidylserine (POPS) and phosphatidylglycerol (POPG), we observed a weak interaction with G i1 and G i3 in neutral lipids phosphatidylethanolamine (POPE) and phosphatidylcholine (POPC) (Fig. 1c, d —G i1 and G i3 with epinephrine stabilizes more mB−β 2 AR in the active conformation than epinephrine alone). This result suggested that negatively charged lipids may repel G i1 and G i3 interaction with β 2 AR. Indeed, we observed that negatively charged CHS decreased mB-β 2 AR-G i3 coupling (Fig. 1e ), supporting our hypothesis that negatively charged lipids inhibit coupling. Since CHS is a nonphysiologic cholesterol analog, we omitted negatively charged CHS in subsequent experiments in order to isolate the effect of phospholipid charge on mB−β 2 AR−G i interactions. Given reports that PKA phosphorylation of β 2 AR increases β 2 AR−G i interaction in vitro [11] , we also tested the effect of PKA phosphorylation, but no enhancement of mB−β 2 AR interaction with G i1 , G i2 , or G i3 was observed (Supplementary Fig. 2 ), suggesting that phosphorylation does not potentiate β 2 AR−G i interaction under our experimental conditions, and that other mechanisms may enhance β 2 AR−G i interaction. In contrast to G i1 and G i3 , we were unable to detect coupling to G i2 in any of the lipid-detergent mixtures (Fig. 1c ), suggesting that the interaction is low affinity. Of interest, G i1 and G i3 share higher sequence identity than either subtype shares with G i2 . To confirm the lack of coupling to G i2 observed by fluorescence analysis, we examined β 2 AR-stimulated G protein turnover of GTP in net neutral DDM + POPC for G i2 and G i3 (Supplementary Fig. 3 ). As expected from our fluorescence studies, we observed robust β 2 AR-induced GTP turnover for G i3 , but only weak β 2 AR-induced GTP turnover for G i2 . In contrast we observed strong coupling of G i2 to purified neurotensin receptor, indicating that the G i2 protein was functional. While both G i2 and G i3 couple to β 2 AR in cardiac myocytes [3] , the coupling efficiency using purified components is substantially different (see Discussion). We therefore focused on β 2 AR−G i3 coupling in further studies. Next we examined how the lipid environment affects β 2 AR activation of G i3 . In the presence of epinephrine, significantly more β 2 AR-induced GTP turnover was detected in DDM micelles containing POPE (net neutral lipid) than in DDM micelles containing POPS (net negative) (Fig. 1f ). This effect on β 2 AR-mediated turnover was significant, even though the lipid:DDM mole ratio was only 1:5. POPE did not increase basal GTP turnover by G i3 in the absence of β 2 AR (Supplementary Fig. 4 ). Taken together, these results indicate that the charge property of phospholipids regulates G i activation by β 2 AR. Ca 2+ facilitates G i3 coupling in negatively charged lipids Ca 2+ , a ubiquitous second messenger, plays an important role in cardiac myocytes; Ca 2+ waves, magnified by G s activation, drive the cardiac myocyte contraction machinery. Recently Ca 2+ was reported to regulate T-cell receptor activation by modulating the charge property of lipids [27] . Given that Ca 2+ interaction with negative charge on phospholipids neutralizes the charge, we tested whether Ca 2+ improves mB−β 2 AR−G i3 coupling efficiency in negatively charged DDM + POPS. Indeed, Ca 2+ improved coupling efficiency in DDM + POPS micelles (Fig. 2a ), and this effect required lipid (Fig. 2b ). Moreover, Ca 2+ had little effect on mB−β 2 AR−G s interaction, implicating differences in G s and G i3 surface charge. Fig. 2 Ca 2+ facilitates G i3 coupling in negatively charged phosphatidylserine. a The effect of 10 mM CaCl 2 on mB−β 2 AR−G protein interaction (G i3 and G s ) was examined in micelles containing 5:1 DDM:POPS (mole ratio). Data were collected in the absence (APO) and presence (100 μM) of epinephrine. mB−β 2 AR concentration is 250 nM. Data are mean ± s.e.m. of three independent experiments. Multiplicity adjusted P values were computed by two-way ANOVA followed by Sidak’s post hoc test between CaCl 2 conditions. b The effect of 10 mM CaCl 2 on mB−β 2 AR−G i3 interaction in DDM micelles ± POPS (i.e. DDM alone vs. 2.5:1 DDM:POPS mole ratio). mB−β 2 AR concentration is 250 nM. Data are mean ± s.e.m. of three independent experiments. Multiplicity adjusted P values were computed by three-way ANOVA followed by Sidak’s post hoc test between indicated groups. Source data are provided in the Source Data File Full size image Ca 2+ interacts with the amino terminal helix of G i3 Next, we sought to determine the mechanism by which Ca 2+ −POPS interactions increase mB−β 2 AR coupling to G i3 but not to G s . Given that the amino terminal helix (αN) of G protein is adjacent to the membrane when coupled to the β 2 AR [25] , and polybasic residues on G s αN are known to facilitate membrane interaction [28] , we looked for a possible selectivity determinant within αN. Since αN of G s and G i are differentially charged (Fig. 3a ), we first replaced αN of G s with αN of G i3 , creating a G i3 -G s chimera (Fig. 3b ). Fig. 3 Ca 2+ interacts with the amino terminal helix of G i3 . a Membrane-facing surfaces of G s and G i1 Ras domains, with β 2 AR shown in gray. The membrane-facing surface of G i1 was modeled by superimposing the Ras domain of G i1 (PDB: 1GP2 [70] ) onto the structure of G s in complex with β 2 AR (PDB: 3SN6 [69] ). Red and blue signify negative and positive charge on G protein, respectively. Dashed lines highlight the region in αN where charge differs: The sequence is KDKQ in WT G s vs. EDGE in WT G i1 (and in G i2 , G i3 ). b mB−β 2 AR−G protein dose−response curves ± 10 mM CaCl 2 . 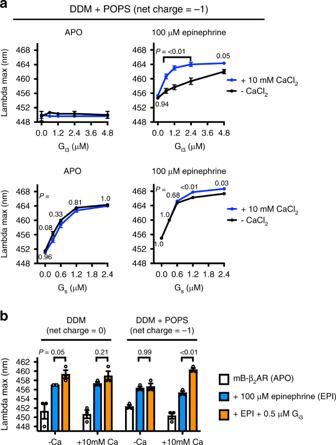Fig. 2 Ca2+facilitates Gi3coupling in negatively charged phosphatidylserine.aThe effect of 10 mM CaCl2on mB−β2AR−G protein interaction (Gi3and Gs) was examined in micelles containing 5:1 DDM:POPS (mole ratio). Data were collected in the absence (APO) and presence (100 μM) of epinephrine. mB−β2AR concentration is 250 nM. Data are mean ± s.e.m. of three independent experiments. Multiplicity adjustedPvalues were computed by two-way ANOVA followed by Sidak’s post hoc test between CaCl2conditions.bThe effect of 10 mM CaCl2on mB−β2AR−Gi3interaction in DDM micelles ± POPS (i.e. DDM alone vs. 2.5:1 DDM:POPS mole ratio). mB−β2AR concentration is 250 nM. Data are mean ± s.e.m. of three independent experiments. Multiplicity adjustedPvalues were computed by three-way ANOVA followed by Sidak’s post hoc test between indicated groups. Source data are provided in the Source Data File Data were generated with the G protein depicted below the curves: mutations were made in αN and corresponding electrostatic models are shown. Epinephrine was not included in experiments titrating G s WT, G i3 -G s Chimera, or G s -neg. to enhance the effect of CaCl 2 . Epinephrine (100 μM) was included in experiments titrating G i3 WT and G i3 -pos. mB−β 2 AR concentration is 250 nM. Data are mean ± s.e.m. of three independent experiments. Multiplicity adjusted P values were computed by two-way ANOVA followed by Sidak’s post hoc test between CaCl 2 conditions. Source data are provided in the Source Data File Full size image While Ca 2+ does not promote mB−β 2 AR coupling to WT G s (Fig. 3b ), it did promote mB−β 2 AR coupling to the G i3 -G s chimera (Fig. 3b ). Next, we compared the membrane-facing charge of G s WT αN and G i3 WT αN. Structural analysis revealed that charge differed at the C terminal end of αN: G i harbors a negatively charged motif (EDGE) at the position where G s harbors a positively charged motif (KDKQ) (Fig. 3a ). To examine whether this motif dictates a differential response to Ca 2+ , we constructed a G s mutant (G s -neg.) containing the negatively charged motif of G i3 (KDKQ → EDGE). Ca 2+ increased mB−β 2 AR interaction with this mutant (Fig. 3b ), suggesting the EDGE motif is responsible for the effect of Ca 2+ on G i3 αN. Taken together, our results imply that Ca 2+ coordinates an interaction between the negatively charged EDGE motif on αN of G i3 and the headgroup of POPS. In the absence of Ca 2+ , like-charge repulsion decreases mB-β 2 AR coupling to G i3 . We also constructed a G i3 mutant (G i3 -pos.) containing the positively charged motif of G s (EDGE → KDKQ). The mutations only partially removed the effect of Ca 2+ (Fig. 3b ), indicating the effect of Ca 2+ on G i3 extends beyond an effect on αN (see Discussion). Bilayer charge differentially affects G s and G i3 coupling Owing to their geometry and charge, phospholipids might induce changes in the size and shape of micelle assemblies which could also influence mB−β 2 AR−G protein interaction [29] , [30] . To examine the effects of phospholipids in a more native environment, and to restrict the size and shape of lipid ensembles, helping us isolate the effect of membrane charge, we reconstituted mB−β 2 AR into nanodisc bilayers and purified the nanodiscs to homogeneity using size-exclusion chromatography (Supplementary Fig. 5 ). First, we compared the influence of lipid composition in the absence of Ca 2+ . Negatively charged bilayers (DOPG and DOPS bilayers), previously reported to increase agonist affinity [14] , expectedly red-shifted the emission spectra of unliganded mB−β 2 AR, suggesting these lipids stabilize an active conformation. Additionally, unliganded mB-β 2 AR and G s could fully couple in negatively charged bilayers but not in neutral bilayers (Fig. 4 ), suggesting negatively charged lipids might facilitate signaling through G s . In contrast, negatively charged lipids (especially DOPS bilayers) decreased G i3 coupling to epinephrine-activated mB−β 2 AR (Fig. 4 ). Fig. 4 Bilayer charge differentially affects G s and G i3 coupling. The effect of G s (left) and G i3 (right) concentration on mB−β 2 AR fluorescence was examined in nanodisc bilayers of varying phospholipid composition (DOPC, DOPE, DOPG, DOPS). Epinephrine was omitted (APO) or included (30 μM). Interaction with G protein is read out as an increase in lambda max. The net charge of the phospholipid is indicated in parentheses. mB−β 2 AR concentration is 100 nM; maximum stoichiometry is 12:1 (for G s ) and 24:1 (for G i3 ). Data are mean ± s.e.m. of three independent experiments. Source data are provided in the Source Data File Full size image In fact, in negatively charged bilayers without epinephrine, G i3 unexpectedly blue-shifted the emission spectra of mB−β 2 AR. While this may indicate that G i3 stabilizes the β 2 AR in an inactive conformation in negatively charged lipids, it may represent a nonspecific interaction of inactive G i3 with the β 2 AR or the lipid bilayer. Cations promote G i3 coupling in negatively charged bilayers Next we examined the effect of Ca 2+ and Mg 2+ . In the absence of G i3 , both Ca 2+ and Mg 2+ reversed the active-state stabilizing effect of negatively charged DOPS and DOPG bilayers (Fig. 5a ). Despite this, Ca 2+ and Mg 2+ increased mB-β 2 AR coupling to G i3 in negatively charged DOPS bilayers, but only Ca 2+ was efficacious at concentrations below 1 mM (Fig. 5a ). Ca 2+ similarly affected mB−β 2 AR−G i3 interaction in negatively charged DOPG bilayers (Fig. 5a ), but the magnitude of the effect in DOPG bilayers was less than observed in DOPS bilayers due to the higher baseline effect of DOPG on β 2 AR conformation. Fig. 5 Ca 2+ and Mg 2+ facilitate G i3 coupling in negatively charged bilayers a The effect of CaCl 2 and MgCl 2 concentration on mB−β 2 AR fluorescence in DOPS and DOPG nanodisc bilayers was examined in the presence and absence of G i3 . Epinephrine was included (30 μM) or omitted (APO). EC 50 is mean ± s.e.m. b The effect of G protein concentration (G i3 and G s ) on mB−β 2 AR fluorescence ± 3 mM CaCl 2 was examined in DOPS nanodiscs in the absence (APO) and in the presence (EPI) of epinephrine (30 μM). c The effect of G i3 on mB−β 2 AR fluorescence ± 3 mM CaCl 2 was examined in DOPE, DOPC, and DOPG nanodisc bilayers in the presence of 30 μM epinephrine (EPI). d The effect of G i2 concentration on mB−β 2 AR fluorescence ± 3 mM CaCl 2 was examined in DOPS nanodisc bilayers in the presence of 30 μM epinephrine (EPI). a – d mB−β 2 AR concentration is 100 nM. The net charge of the phospholipid molecule is indicated in parentheses. Data are mean ± s.e.m. of three independent experiments. Source data are provided in the Source Data File Full size image We also compared the effect of Ca 2+ on mB−β 2 AR interactions with G protein subtypes (G s versus G i3 ) in DOPS bilayers. As observed in micelles, Ca 2+ increased mB−β 2 AR coupling to G i3 but not to G s (Fig. 5b ). Ca 2+ also improved mB−β 2 AR−G i3 coupling efficiency in negatively charged DOPG bilayers (Fig. 5c ). However, incorporating Ca 2+ did not enable detection of mB−β 2 AR interaction with the G i2 subtype of G i (Fig. 5d , see Discussion). While Ca 2+ interacts with net negative PS and PG with relatively high affinity, it also interacts with the negatively charged phosphate group on net neutral PC [31] and PE lipids [31] , [32] . In neutral DOPE and DOPC bilayers (Fig. 5c and Supplementary Fig. 6 ), Ca 2+ only slightly enhanced mB−β 2 AR−G i3 interaction, which could be attributable to weaker Ca 2+ /DOPE and Ca 2+ /DOPC interactions that have been reported. Taken together, our observations provide biochemical evidence that local membrane charge can regulate β 2 AR−G protein interaction. We observed that local membrane charge regulates β 2 AR−G protein interaction. Negatively charged membrane promotes β 2 AR−G s coupling and suppresses β 2 AR−G i3 coupling. 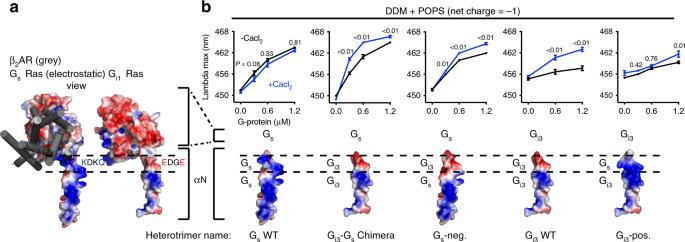Fig. 3 Ca2+interacts with the amino terminal helix of Gi3.aMembrane-facing surfaces of Gsand Gi1Ras domains, with β2AR shown in gray. The membrane-facing surface of Gi1was modeled by superimposing the Ras domain of Gi1(PDB: 1GP270) onto the structure of Gsin complex with β2AR (PDB: 3SN669). Red and blue signify negative and positive charge on G protein, respectively. Dashed lines highlight the region in αN where charge differs: The sequence is KDKQ in WT Gsvs. EDGE in WT Gi1(and in Gi2, Gi3).bmB−β2AR−G protein dose−response curves ± 10 mM CaCl2. Data were generated with the G protein depicted below the curves: mutations were made in αN and corresponding electrostatic models are shown. Epinephrine was not included in experiments titrating GsWT, Gi3-GsChimera, or Gs-neg. to enhance the effect of CaCl2. Epinephrine (100 μM) was included in experiments titrating Gi3WT and Gi3-pos. mB−β2AR concentration is 250 nM. Data are mean ± s.e.m. of three independent experiments. Multiplicity adjustedPvalues were computed by two-way ANOVA followed by Sidak’s post hoc test between CaCl2conditions. Source data are provided in the Source Data File However, G s bias is reduced in neutral membrane and in negatively charged membrane in the presence of divalent cations (see model in Fig. 6 ). Fig. 6 Membrane charge is a tunable modulator of β 2 AR−G protein interaction. Models depict epinephrine-bound β 2 AR. Left: In negatively charged lipids, β 2 AR−G s coupling is efficient, but β 2 AR−G i3 coupling is relatively inefficient, in part because β 2 AR−G i3 attraction is countered by membrane-G i3 repulsion. Specifically, negatively charged lipids repel the negatively charged EDGE motif found on the amino terminal helix of G i3 (shown in red), a region that is positively charged in G s (shown in blue). Right: Two mechanisms that neutralize membrane charge facilitate β 2 AR coupling to G i3 . These mechanisms may play a role in G s -to-G i switching in cardiac myocytes. Top right: Ca 2+ and Mg 2+ stabilize a like-charge interaction between the membrane and the EDGE motif. (Note that the effect of Ca 2+ and Mg 2+ may extend beyond an effect on αN positioning.) Bottom right: Epinephrine-stimulated β 2 AR traffics to membrane without negatively charged lipids Full size image We have begun to explore the mechanism by which Ca 2+ increases mB−β 2 AR coupling to G i3 in phospholipids. The effect of Ca 2+ was largely dependent on charged groups on G i3 , indicating Ca 2+ doesn’t simply affect membrane structure. Although G proteins are membrane tethered via lipidation, the lipid anchor of G i3 is not sufficient for optimal interaction with β 2 AR in negatively charged bilayers, possibly due to repulsion of the carboxyl terminal end of the αN helix. We propose that Ca 2+ helps orient the carboxyl terminal end of the αN helix of G i3 near the membrane, thereby facilitating β 2 AR−G i3 interactions. More specifically, we propose that Ca 2+ facilitates the interaction of lipid with the negatively charged EDGE motif on the αN helix of G i3 . Ca 2+ may coordinate a like-charge interaction between the carboxylate groups on the G i3 EDGE motif and the phosphate group present on all lipids. In addition, Ca 2+ may especially stabilize EDGE interaction with PS lipids by coordinating a like-charge interaction between the carboxylate groups on the G i3 EDGE motif and the carboxylate group on PS (not present on PG) (refer to structures in Fig. 1b ), or Ca 2+ might coordinate an intramolecular interaction between the phosphate group and the carboxylate group on PS, freeing the amino group (NH 3 + ) on PS to interact with the carboxylate groups on G i3 . We have previously shown that negatively charged lipids, particularly PG, stabilize the β 2 AR in an active-like conformation as revealed by changes in mB−β 2 AR fluorescence and an increased affinity for agonists [14] . These effects are likely due to interactions between the lipids and positively charged amino acids on the β 2 AR. Here we observed that the effect of DOPG and DOPS on mB-β 2 AR can be reversed by both Ca 2+ and Mg 2+ (Fig. 5a ). Yet, these divalent cations do not appear to reduce coupling to G s . β 2 AR signals from caveolin-rich rafts [33] , [34] within T-tubules [19] . While β 2 AR preferentially interacts with PG in insect cell membrane [14] , the phospholipid composition immediately adjacent to β 2 AR in T-tubules, and how it changes during β 2 AR trafficking, is currently unknown. Net-neutral PC and PE are the major phospholipids in T-tubules [35] , [36] , [37] . However, negatively charged PS is enriched in T-tubules relative to other membrane fractions (7.5−12.3% of total phospholipid) [35] , [36] , [37] , [38] , [39] . While cytosolic Ca 2+ concentrations are typically less than 1 mM [40] , concentrations of Ca 2+ in the mM range may be observed in cardiac myocytes. Investigators have long speculated about the functional role of Ca 2+ in the cleft between the T-tubule membrane (where β 2 AR is localized) and the juxtaposed sarcoplasmic reticulum (SR) [21] , [22] , [41] . During each action potential, extracellular Ca 2+ flows into the cleft through L-type Ca 2+ channels (LTCCs) on the plasma membrane and through ryanodine receptors (RyRs) on the sarcoplasmic reticulum [40] . Cleft Ca 2+ concentrations spark to >100 μM in the absence of epinephrine and >1 mM [42] , [43] following epinephrine stimulation, a consequence of G s activation. Computational models show that negatively charged phospholipids buffer approximately half the Ca 2+ released into the cleft [42] , and experiments have shown that 80% of inner-leaflet bound Ca 2+ is bound to negatively charged phospholipids [44] . Additionally, biochemical investigations show that Ca 2+ can cluster negatively charged PS [45] and PIP 2 [46] , [47] lipids. β 1 AR and β 2 AR signaling through G s alters calcium handling in the cardiac myocyte, and increases the magnitude of Ca 2+ currents and Ca 2+ transients, which stimulate cardiac contraction [40] , [48] . However, elevated Ca 2+ concentrations also activate the Ca 2+ /calmodulin-dependent protein kinase II (CaMKII), which promotes apoptosis, and is implicated in structural remodeling that ultimately results in cardiac dysfunction [9] , [49] , [50] , [51] , [52] . Elevated Ca 2+ also activates calcineurin, which exacerbates pathological hypertrophy [21] . For these reasons, β 1 AR-selective (and nonselective) beta blockers have proven to be efficacious medicines for treatment of heart failure [53] . However, β 2 AR, owing to its dual G s /G i selectivity, is functionally distinct from the strictly G s -coupled β 1 AR, and several lines of evidence suggest β 2 AR−G i signaling functions to keep G s signaling in check via negative feedback: β 2 AR−G i signaling occurs minutes after β 1 AR−G s and β 2 AR−G s signaling [2] , β 2 AR−G i signaling suppresses changes in calcium handling [48] , [54] , and β 2 AR−G i signaling is antiapoptotic [7] , [8] . While the mechanism that triggers β 2 AR−G i signaling is unknown, our biochemical observations suggest elevated Ca 2+ concentrations could trigger β 2 AR coupling to G i3 . It is notable that overexpression of the Ca 2+ /sodium exchanger facilitates β 2 AR−G i suppression of β 1 AR−G s signaling [55] , and overexpression has been cited to increase the inward LTCC Ca 2+ current [56] . It is also notable that intracellular Ca 2+ [57] , [58] and Mg 2+ [58] concentrations rise during ischemia and rise even higher during reperfusion. Whether the rising concentrations facilitate β 2 AR-G i signaling is unknown. However, β 2 AR−G i signaling can reduce the extent of cardiac necrosis caused by ischemia and reperfusion [59] . We were surprised that we did not observe mB−β 2 AR coupling to G i2 under conditions where we observed coupling to G i1 and G i3 (Fig. 1c , Supplementary Fig. 3 ). Although G i2 contains the αN EDGE motif, we did not observe mB−β 2 AR−G i2 interaction in the presence of Ca 2+ (Fig. 5d ). While the sequences of Gα i1 and Gα i3 are 94% identical, Gα i2 shares less sequence identity with Gα i1 and Gα i3 , 88% and 86%, respectively. Supplementary Fig. 7 shows the location of the amino acid differences in G i2 relative to both G i1 and G i3 using the recent cryo-electron microscopy structure of the adenosine A1-G i2 complex (PDB: 6D9H [60] ). It can be seen that these amino acids do not appear to interact directly with the receptor in the nucleotide-free complex. However, these amino acids may form weak interactions with the poorly ordered intracellular loop 3 that is not observed in the structure, or may interact with other domains of the receptor during complex formation. Previous studies provide evidence for at least one transient intermediate state in formation of the β 2 AR−G s complex [61] . Both G i2 and G i3 couple to β 2 AR in cardiac myocytes [3] . However, during heart failure, G i2 expression is commonly upregulated [62] , [63] , [64] . In contrast, G i3 upregulation, while reported [65] , is less commonly observed. How selective G i2 upregulation influences β 2 AR−G i signaling is not fully understood. Signaling through G i2 and G i3 could play different roles in cardiac physiology. It is possible that β 2 AR coupling to G i3 plays a role in preventing myocyte damage during transient ischemia or prolonged periods of adrenergic stimulation, such as during exercise. Both of these conditions would be associated with elevated cytosolic Ca 2+ . In contrast, β 2 AR coupling to G i2 may play a more prominent role in the failing heart. G proteins are a large superfamily, grouped into four subfamilies (G s , G i/o , G q/11 , G 12/13 ) encoded by 16 different genes [66] . Each subfamily activates distinct signaling pathways, and functional effects are cell-type specific. Most GPCRs can signal through more than one G protein subfamily, and ongoing research attempts to identify mechanisms that regulate G protein selectivity within a cell [66] . Whether local membrane charge affects G i interaction with other G i -coupled GPCRs is not currently known. In cardiac myocytes, β 2 AR signals from a PS-enriched, Ca 2+ -enriched microenvironment, which highlights the potential relevance of our biochemical observations. Additionally, the observation that Ca 2+ sensing receptor (CaSR) switches from G q to G i after cytosolic Ca 2+ increases [67] is also potentially relevant to our findings. However, knowledge that Ca 2+ facilitates G i interaction with membrane is not sufficient to predict how Ca 2+ might affect G i interaction with other receptors. In conclusion, we show that local membrane charge differentially modulates β 2 AR interaction with competing G protein subtypes (G s and G i ). This discovery expands our knowledge of mechanisms that regulate the G protein coupling selectivity of GPCRs. G protein expression and purification All G proteins were human heterotrimeric G proteins (Gα, Gβ 1 , Gγ 2 ). The Gβ 1 subunit contained an N-terminal 6xHis tag followed by a rhinovirus 3C protease site used for purification [61] . Gα s was the short splice variant. The G i3 -G s chimera was created starting with Gα s , replacing residues 1−38 (the αN helix) with the equivalent region of Gα i3 (residues 1−31 of Gα i3 ) [68] . G s -neg. was a G s mutant with residues 32−35 of Gα s (KDKQ) replaced with the equivalent region in Gα i3 (EDGE). G i3 -pos. was a G i3 mutant with residues 25−28 of Gα i3 (EDGE) replaced with the equivalent region in Gα s (KDKQ). G protein was expressed in Tni insect cells (Expression Systems Cat. 94-002S) using two recombinant baculoviruses, a virus encoding Gα and a separate virus encoding both the Gβ 1 and Gγ 2 subunits. Following infection, cells were incubated for 48 h at 27 °C, harvested by centrifugation, and suspended in lysis buffer (10 mM Tris (pH 7.5), 100 μM MgCl 2 , 5 mM β-mercaptoethanol (BME), 10 μM GDP, and protease inhibitors). The membrane fraction was collected by centrifugation and solubilized using a Dounce homogenizer and buffer comprised of 20 mM HEPES (pH 7.4), 100 mM NaCl, 1% sodium cholate, 0.05% n -dodecyl-β- d -maltopyranoside (DDM), 5 mM MgCl 2 , 5 mM BME, 10 μM GDP, and protease inhibitors. The soluble fraction was isolated by centrifugation, G protein was captured on Sepharose Fast Flow (GE Healthcare) charged with nickel, and gradually exchanged into SEC buffer (20 mM HEPES (pH 7.4), 100 mM NaCl, 0.05% DDM, 100 μM TCEP, 10 μM GDP, 1 mM MgCl 2 ). 3C protease was added to cleave G protein off the resin, and the G protein was dephosphorylated using calf intestinal alkaline phosphatase, antarctic phosphatase, and lambda protein phosphatase. Subsequently, G protein was isolated in SEC buffer using a Superdex 200 10/300 GL column (GE Healthcare). The main peak corresponding to heterotrimeric G protein was collected, concentrated, and frozen. Receptor expression, purification, and labeling The β 2 AR construct was PN1 [14] , where human WT β 2 AR (R16, Q27 variant) is modified to contain an N-terminal FLAG tag, a C-terminal rho-1D4 tag, a TEV protease cleavage site between V24 and T25, and a 3C protease cleavage site between G365 and Y366. Additionally, mutations were introduced to increase expression (M96T, M98T), to remove a glycosylation site (N187E) and to remove reactive cysteines (C378A, C406A). β 2 AR was expressed in Sf9 insect cells (Expression Systems Cat. 94-001S) using recombinant baculovirus and media supplemented with 1 μM alprenolol. Cells expressing β 2 AR were harvested by centrifugation and suspended in lysis buffer (10 mM HEPES (pH 7.4), 1 mM EDTA, 1 μM alprenolol, and protease inhibitors). The membrane fraction was collected by centrifugation and solubilized using a Dounce homogenizer and buffer comprised of 20 mM HEPES (pH 7.4), 100 mM NaCl, 1% n -dodecyl-β- d -maltopyranoside (DDM), 0.03% CHS, 2 mM MgCl 2 , 1 μM alprenolol, and protease inhibitors. The soluble fraction was isolated by centrifugation and anti-FLAG (ATCC HB-9259) affinity chromatography was used to purify β 2 AR, remove alprenolol, and adjust detergent concentration (to 0.1% DDM, 0.01% CHS). Monobromobimane (mB, Thermo Fisher Scientific) labeling was then performed overnight with excess mB in the presence of 100 μM TCEP and the reaction was quenched with 5 mM l -cysteine before further purification. All β 2 AR preparations were functionally purified by alprenolol-Sepharose affinity chromatography and washed on an anti-FLAG column to remove ligand. The eluted β 2 AR was dialyzed in buffer comprised of 20 mM HEPES (pH 7.4), 100 mM NaCl, 0.1% DDM, and 0.02% CHS, concentrated, and dephosphorylated using lambda protein phosphatase. For experiments assessing phosphorylation, unphosphorylated β 2 AR was phosphorylated with protein kinase A in the presence of 2 mM ATP. β 2 AR was stored frozen. Phosphorylation was assessed using the Pro-Q Diamond Phosphoprotein Gel Stain (ThermoFisher Scientific), per the manufacturer’s instructions. Stained acrylamide gels were scanned with a Typhoon 9410 Imager (GE Healthcare). Recombinant human NTSR1 (residues 20−418) contained an A85 1.54 L mutation to increase expression. NTSR1 was purified from Sf9 insect cells into buffer comprised of 20 mM HEPES (pH 7.5), 100 mM NaCl, 5% glycerol, 0.01% lauryl maltose neopentyl glycol (LMNG), 0.001% CHS, and 0.5 µM JMV 449, and stored frozen. Ligands (−) epinephrine was purchased from Sigma (purity > 99%). JMV 449 was purchased from Tocris (purity 97.6%). Micelle composition n -dodecyl-β- d -maltopyranoside (DDM), cholesteryl hemisuccinate (CHS), and 1-palmitoyl-2-oleoyl-sn-glycero-3-(PE,PC,PG,PS) lipids (Avanti Polar Lipids) were mixed in the indicated ratios and solubilized in chloroform. Chloroform was evaporated, and the films were re-suspended in 20 mM HEPES (pH 7.4), 100 mM NaCl. Fluorescence spectroscopy In experiments examining mB-β 2 AR in micelles, mB−β 2 AR was preincubated (30 min room temperature) in micelle stock prior to dilution with other reaction components. pH 7.4 HEPES buffer (containing 100 mM NaCl, ± ligand, ± CaCl 2 or MgCl 2 ) and G protein were sequentially included. Mixtures were incubated 2.5–3.0 h at room temperature. Final mB−β 2 AR concentration was 100−300 nM. Emission spectra were read at 22 °C using a Fluorolog-3 spectrofluorometer (Horiba Jobin Yvon Inc.). (Bandpass = 4 nm; Excitation = 370 nm; Emission = 420−500 nm, collected in 1 nm increments). The raw S1c/R1c spectra were smoothed using Prism (GraphPad Software) ( n = 15 neighbors, second-order polynomial). Lambda max is defined as the wavelength at which fluorescence emission is maximum. To determine the EC 50 , data were fit to the agonist vs. response model in Prism 7.0d software. GTP turnover Where lipid environments were compared, samples were prepared as they were for fluorescence spectroscopy. Following β 2 AR incubation with G protein, 1 μM GTP + 5 μM GDP mixtures (final concentration) were added to initiate the GTP turnover reaction. Reaction buffer contained 20 mM HEPES (pH 7.4) and 100 mM NaCl. Where G i2 and G i3 were compared, the GTP turnover reaction was initiated by mixing a solution containing 10 μM GTP and ligand-bound receptor (4 μM β 2 AR + 800 μM epinephrine or 1 μM NTSR1 + 10 μM JMV 449) in equal volume with a solution containing 2.5 μM G protein, 20 μM GDP, 20 mM MgCl 2 , and 200 μM TCEP. At the indicated timepoints, the GTP remaining was assessed using the GTPase-Glo assay (Promega), which detects GTP using a luminescence readout. Luminescence was detected using a SpectraMax Paradigm plate reader equipped with a TUNE SpectraMax detection cartridge (Molecular Devices). Background luminescence was subtracted from experimental reactions. Statistics Two-way and three-way ANOVA were performed using Graphpad Prism 7.0d. Electrostatic modeling Structural views and mutant models were generated using PyMOL (Schrödinger, LLC). We selected rotomer positions that most closely matched those seen in PDB 3SN6 [69] (for the G i3 -pos. model) and PDB 1GP2 [70] (for the G s -neg. model). Continuum electrostatics models were calculated using the APBS [71] plugin (MG Lerner, University of Michigan, Ann Arbor) for PyMOL. Atomic charge and radii were calculated using the online PDB2PQR server [72] (pH 7.4, PARSE force field, hydrogen bond optimization, clash avoidance). Nanodisc reagents 1,2-dioleoyl-sn-glycero-3-(PE,PC,PG,PS) lipids (Avanti Polar Lipids) were used because of their low phase transition temperature. Lipids were dissolved in buffer comprised of 20 mM HEPES (pH 7.5), 100 mM NaCl, 50 mM sodium cholate, 1 mM EDTA at 16.6 mM, and were sonicated on ice before use. The MSP belt was MSP1E3D1 [73] . pMSP1E3D1 was a gift from Stephen Sligar (Addgene plasmid #20066). The protein was expressed in BL21(DE3) E. coli (Cat. 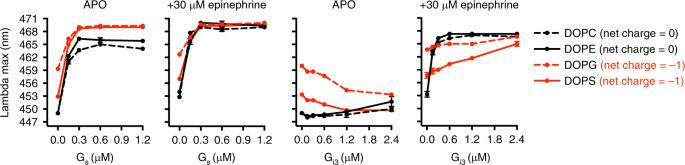Fig. 4 Bilayer charge differentially affects Gsand Gi3coupling. The effect of Gs(left) and Gi3(right) concentration on mB−β2AR fluorescence was examined in nanodisc bilayers of varying phospholipid composition (DOPC, DOPE, DOPG, DOPS). Epinephrine was omitted (APO) or included (30 μM). Interaction with G protein is read out as an increase in lambda max. The net charge of the phospholipid is indicated in parentheses. mB−β2AR concentration is 100 nM; maximum stoichiometry is 12:1 (for Gs) and 24:1 (for Gi3). Data are mean ± s.e.m. of three independent experiments. Source data are provided in the Source Data File 70235-3 Millipore Sigma), and cells were lysed with sonication in 10 mM Tris-HCl, 100 mM NaH 2 PO 4 , 6 M GuHCl, 1% Triton X-100 (pH 8.0). The soluble fraction was isolated by centrifugation and passed through a Sepharose Fast Flow (GE Healthcare) column charged with nickel. Immobilized protein was washed with buffer comprised of 10 mM Tris-HCl, 100 mM NaH 2 PO 4 , 6 M GuHCl, and 0.2% Triton X-100 (pH 7.0), and then washed with buffer comprised of 50 mM NaH 2 PO 4 , 300 mM NaCl, and 0.2% Triton X-100 (pH 8.0). The protein was eluted using 250 mM imidazole. 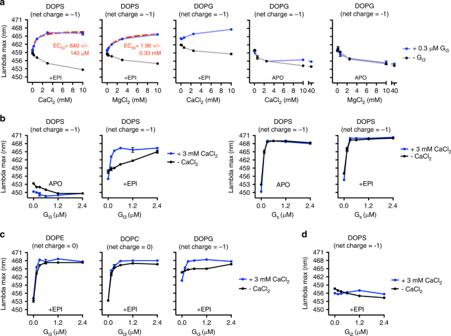Fig. 5 Ca2+and Mg2+facilitate Gi3coupling in negatively charged bilayersaThe effect of CaCl2and MgCl2concentration on mB−β2AR fluorescence in DOPS and DOPG nanodisc bilayers was examined in the presence and absence of Gi3. Epinephrine was included (30 μM) or omitted (APO). EC50is mean ± s.e.m.bThe effect of G protein concentration (Gi3and Gs) on mB−β2AR fluorescence ± 3 mM CaCl2was examined in DOPS nanodiscs in the absence (APO) and in the presence (EPI) of epinephrine (30 μM).cThe effect of Gi3on mB−β2AR fluorescence ± 3 mM CaCl2was examined in DOPE, DOPC, and DOPG nanodisc bilayers in the presence of 30 μM epinephrine (EPI).dThe effect of Gi2concentration on mB−β2AR fluorescence ± 3 mM CaCl2was examined in DOPS nanodisc bilayers in the presence of 30 μM epinephrine (EPI).a–dmB−β2AR concentration is 100 nM. The net charge of the phospholipid molecule is indicated in parentheses. Data are mean ± s.e.m. of three independent experiments. Source data are provided in the Source Data File 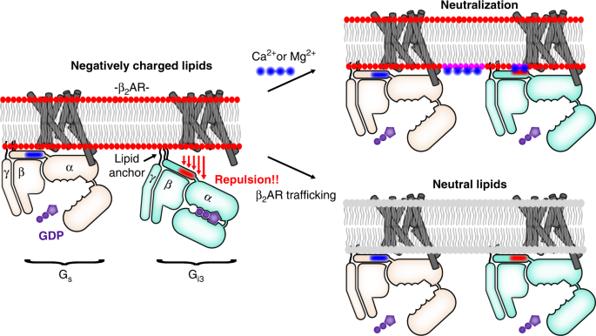Fig. 6 Membrane charge is a tunable modulator of β2AR−G protein interaction. Models depict epinephrine-bound β2AR. Left: In negatively charged lipids, β2AR−Gscoupling is efficient, but β2AR−Gi3coupling is relatively inefficient, in part because β2AR−Gi3attraction is countered by membrane-Gi3repulsion. Specifically, negatively charged lipids repel the negatively charged EDGE motif found on the amino terminal helix of Gi3(shown in red), a region that is positively charged in Gs(shown in blue). Right: Two mechanisms that neutralize membrane charge facilitate β2AR coupling to Gi3. These mechanisms may play a role in Gs-to-Giswitching in cardiac myocytes. Top right: Ca2+and Mg2+stabilize a like-charge interaction between the membrane and the EDGE motif. (Note that the effect of Ca2+and Mg2+may extend beyond an effect on αN positioning.) Bottom right: Epinephrine-stimulated β2AR traffics to membrane without negatively charged lipids Impurities were precipitated by two rounds of heating at 70 °C for 1 h; after each round, the soluble fraction was isolate by centrifugation. The final soluble fraction containing MSP1E3D1 was supplemented with 20 mM sodium cholate and purified further using a HiPrep 16/60 Sephacryl S-300 HR size-exclusion column (GE Healthcare) equilibrated with buffer comprised of 20 mM HEPES, 100 mM NaCl, 1 mM EDTA, and 20 mM sodium cholate. The main peak corresponding to MSP1E3D1 was collected, dialyzed in 20 mM HEPES, 100 mM NaCl, 1 mM EDTA, 5 mM sodium cholate, concentrated to 728 μM, and frozen. Nanodisc reconstitution Nanodiscs were formed with one lipid type (i.e. 100% DOPS, DOPG, DOPE, or DOPC). Reconstitution was initiated by sequentially mixing water, 20× reconstitution buffer (400 mM HEPES (pH 7.5), 2 M NaCl, 20 mM EDTA), lipid, mB−β 2 AR, and MSP1E3D1. The volume of mB−β 2 AR stock added to the mixture was ~13% of the final mixture volume. MSP1E3D1 and mB−β 2 AR were added 1:10 (molar ratio). Lipid and MSP1E3D1 were added 35:1 (molar ratio). The mixture was incubated at 4 °C for 2 h. Subsequently, Bio-Beads SM-2 resin (107.1 mg per μmol lipid, Bio-Rad) were added (4 °C for 4 h) to remove detergent, which triggers the reconstitution of mB−β 2 AR in nanodisc bilayers. The soluble fraction was isolated by centrifugation. Bare nanodiscs were separated from nanodiscs containing mB−β 2 AR using anti-FLAG (ATCC HB-9259) affinity chromatography. The eluate was incubated with 5 mM EDTA at 4 °C for ≥ 1.5 h to remove divalent cations. Subsequently, samples were injected into a Superdex 200 10/300GL size-exclusion column (GE Healthcare) equilibrated in buffer comprised of 20 mM HEPES (pH 7.4), 100 mM NaCl, and the main peak corresponding to nanodisc mB−β 2 AR was harvested, concentrated, and frozen. The concentration of nanodisc mB−β 2 AR was approximated by SDS-PAGE, using detergent solubilized β 2 AR as a protein concentration reference standard. Reporting summary Further information on research design is available in the Nature Research Reporting Summary linked to this article.